Total synthesis of feglymycin based on a linear/convergent hybrid approach using micro-flow amide bond formation Feglymycin is a naturally occurring, anti-HIV and antimicrobial 13-mer peptide that includes highly racemizable 3,5-dihydroxyphenylglycines (Dpgs). Here we describe the total synthesis of feglymycin based on a linear/convergent hybrid approach. Our originally developed micro-flow amide bond formation enabled highly racemizable peptide chain elongation based on a linear approach that was previously considered impossible. Our developed approach will enable the practical preparation of biologically active oligopeptides that contain highly racemizable amino acids, which are attractive drug candidates. Biologically active peptides have garnered considerable attention as drug candidates because their target specificity is generally higher than that of small molecule-based drugs, and their production cost is lower than that of protein-based drugs [1] , [2] , [3] . In particular, oligopeptides consisting of <20 amino acids account for three-fourths of existing marketed peptide drugs [3] . Therefore, efficient and practical synthesis of these oligopeptides is highly important. In general, a linear/convergent hybrid approach is used for the synthesis of these oligopeptides: (1) short peptides (<10 amino acids) are prepared based on a linear strategy wherein peptide chains are elongated one-by-one. This linear strategy enables the facile installation of various amino acids for rapid analogue synthesis, and it minimizes the protecting group manipulation of terminal carboxylic acids while avoiding undesired diketopiperazine formation; and (2) the prepared short peptides are coupled in a convergent manner to afford the target oligopeptides because longer peptides are often poorly soluble against solvents. In addition, this approach facilitates purification because the molecular weight of the desired oligopeptides is much different from that of their precursors. Many arylglycine-containing biologically active oligopeptides have been reported, and they are highly important as drugs and drug candidates. Phenylglycine (Phg), 4-hydroxyphenylglycine (Hpg) and 3,5-dihydroxyphenylglycine (Dpg) are the most important representatives of the arylglycines because they can be found in various biologically active natural products such as formadicin, ramoplanin, vancomycin and teicoplanin [4] . These arylglycines significantly contribute to the biological activity of these natural products [4] . Despite their importance, synthetic methodologies that can be used for arylglycines-containg oligopeptides is very limited due to their racemization-prone nature. Reportedly, phenylglycine is 60 times more prone to racemization than alanine [5] . Dpg is even more racemization-prone than the phenylglycine [4] . Feglymycin isolated from Streptomyces sp. DSM 11171 (refs 6 , 7 ) is a biologically active oligopeptide composed of 13 amino acids involving Hpgs and highly racemizable Dpgs. The biological activity of feglymycin involves strong anti-HIV activity [8] and moderate antimicrobial activity [9] , [10] , and its unique helical conformation [11] makes it an attractive lead compound for drug development. In 2009, the Süssmuth group reported the first total synthesis of feglymycin based on a highly convergent approach, in which D -Dpgs were coupled with the neighbouring C-terminal side of amino acids at an initial stage [12] . This amidation of the D -Dpgs with amino acids was performed using a coupling agent, 3-(diethyloxyphosphoryloxy)-1,2,3-benzotriazin-4(3 H )-one (DEPBT). Then, the resultant dipeptides/tripeptides were coupled to afford hexapeptide and heptapeptide. The DEPBT was crucial to avoid an undesired racemization reaction. A linear approach to the syntheses of the hexapeptide and the heptapeptide would have previously described merits. However, the Süssmuth group reported that the coupling of D -Dpgs with longer peptides based on a linear approach resulted in severe racemization of the D -Dpgs and provided an inseparable mixture of diastereomers even when using DEPBT. The Süssmuth group concluded that a linear approach for the hexapeptide and the heptapeptide containing D -Dpgs was not possible [12] . The development of peptide chain elongation based on a linear approach is important not only for the synthesis of feglymycin and related compounds, but also for the synthesis of other arylglycines-containg biologically active oligopeptides. Recent marked progress in micro-flow technology [13] , [14] , [15] , [16] , [17] , [18] , [19] , [20] has enabled precise control of the reaction time (<1 s) and temperature [21] , [22] , [23] . We have studied micro-flow acylations [24] , [25] and recently reported micro-flow amide bond formation using a high atom economy and an inexpensive coupling agent, triphosgene [26] . We envisaged that if micro-flow amide bond formation enables the amidation of Dpgs without severe racemization, then it should be possible to use a linear synthetic approach to prepare the hexapeptide and the hepapeptide. Herein, we wish to report the total synthesis of feglymycin based on a linear/convergent hybrid synthetic approach using a micro-flow amide bond formation that suppresses the undesired racemization. In detail, we planned to couple the hexapeptide and the heptapeptide in a convergent manner for the total synthesis of feglymycin and synthesize both oligo peptides based on a linear approach using micro-flow amide bond formation. The challenge was to suppress any undesired racemization of the highly racemizable Dpgs using our micro-flow amidation. 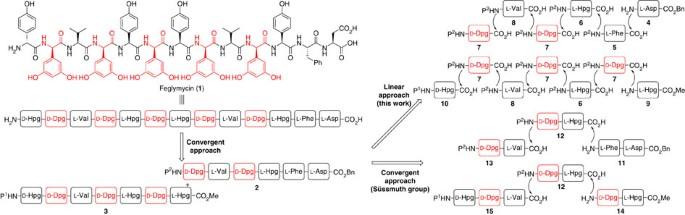Figure 1: Synthetic strategy for feglymycin (1). Our linear synthetic approach and Süssmuth’s convergent synthetic approaches. Süssmuth concluded that the linear approach for oligopeptides2and3containingD-Dpgs was not possible. Examination of micro-flow amide bond formation of arylglycines The key micro-flow amide bond formation of arylglycines was examined using readily available D -Hpgs 10 and 16 ( Table 1 ). We connected two T-shaped mixers with Teflon tubing and immersed them in a water bath. A solution of carboxylate 10 in solvent A was introduced into the first mixer with a syringe pump. The solution of triphosgene in MeCN was also introduced into the first mixer with a syringe pump to rapidly generate symmetric anhydride in situ [26] (<0.5 s). To accomplish amidation (<4.3 s), a solution of amine 16 in solvent B was then introduced into the second mixer with a syringe pump. The reaction was quenched by pouring the mixture into a saturated aqueous solution of NH 4 Cl, brine and ethyl acetate (micro-flow reactor setup, see Supplementary Methods ). To investigate the influence of the protecting group on a nitrogen atom (=P), three protecting groups were examined ( Table 1 ): t- butoxycarbonyl (Boc), 10a ; benzyloxycarbonyl (Cbz), 10b ; and, allyloxycarbonyl (Alloc), 10c . The 9-fluorenylmethoxycarbonyl (Fmoc) group was not examined because we feared that the basic deprotection conditions might cause undesired racemization. We did not protect the phenolic hydroxyl group (p K a = ca . 10) in D -Hpgs 10 because we did not expect the carboxylate generated from an equimolar amount of N,N -diisopropylethylamine (DIEA) and D -Hpg (p K a of CO 2 H in D -Hpg= ca. 2) to deprotonate the phenolic hydroxyl group in D -Hpg to afford an undesired highly nucleophilic phenoxide. On the other hand, the nucleophilicity of neutral phenolic hydroxyl group is much lower than that of an amino group, and, therefore, we speculated that the undesired nucleophilic attack of the phenolic hydroxyl group would not occur. In our previous report, N,N -dimethylformamide (DMF) and MeCN were used for solvents A and B, respectively [26] . However, carboxylate 10a and amine 16 were not soluble against these solvents. Therefore, N,N -dimethylacetoamide (DMA) was used instead of DMF and MeCN (entries 1–5). Carboxylates 10b (P=Cbz) and 10c (P=Alloc) afforded the desired products 18b and 18c in good yields (entries 2 and 3), respectively, whereas 10a (P=Boc) afforded 18a in a low yield (entry 1). To suppress racemization, the reaction was carried out at 10 °C. As expected, the generation of undesired epimers 19b and 19c was suppressed (entries 4 and 5), although a slight decrease in yield was observed in the case of carboxylate 10b (entry 2 versus 4). The use of H 2 O/MeCN for solvent B improved the yield of 18b in the case of carboxylate 10b (P=Cbz) without increasing racemization (entry 4 versus 6). On the other hand, in the case of 10c (P=Alloc), comparable results were observed (entry 5 versus 7). The corresponding batch reaction resulted in increased racemization (entry 7 versus 8). The use of N -methylpyrrolidone (NMP) and N , N′ -dimethylpropyleneurea (DMPU) that could dissolve 10c resulted in a decrease in the yields (entries 9 and 10). Entries 5 ( condition A ) and 7 ( condition B ) were used for the coupling of arylglycines retaining an Alloc group, and entry 6 (condition C) was used for the coupling of arylglycine retaining a Cbz group in the following peptide chain elongations. We decided to use the Cbz group for P 1 and the Alloc group for P 2 ( Fig. 1 ) because the Cbz group could be removed along with the benzyl (Bn) group under hydrogenolysis conditions. Table 1 Micro-flow amide bond formation of D -Hpgs 10 and 16. Full size table Figure 1: Synthetic strategy for feglymycin (1). Our linear synthetic approach and Süssmuth’s convergent synthetic approaches. Süssmuth concluded that the linear approach for oligopeptides 2 and 3 containing D -Dpgs was not possible. Full size image Synthesis of C-terminal hexapeptide 2 We started with a synthesis of the C-terminal dipeptide 20 ( Fig. 2 ). Micro-flow amide bond formation afforded a mixture of 5 , 20 and the HCl salt of DIEA. The desired dipeptide 20 was readily isolated via simple aqueous workup and recrystallization (70% yield, 13 g). Salt-free carboxylic acid 5 was also recovered in a pure form (63% based on unreacted 5 ) via simple aqueous workup and recrystallization. 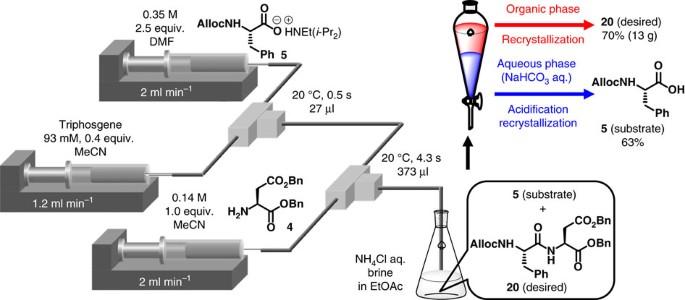Figure 2: Micro-flow synthesis of dipeptide 20. Dipeptide20was prepared by micro-flow amide bond formation. The obtained dipeptide was readily purified via simple aqueous workup and recrystallization. Figure 2: Micro-flow synthesis of dipeptide 20. Dipeptide 20 was prepared by micro-flow amide bond formation. The obtained dipeptide was readily purified via simple aqueous workup and recrystallization. Full size image Peptide chain elongation was performed based on the linear approach, as shown in Fig. 3 . First, an Alloc group was removed from the protected dipeptide 20 under neutral conditions [27] , [28] , [29] using a batch reactor. Micro-flow amidation with carboxylate 6 was performed under condition A with slight modification (activation time: 1.0 s), because dipeptide 11 was not dissolved in the H 2 O/MeCN mixed solvent with the use of condition B . After recrystallization, the desired pure tripeptide 21 , which did not contain an epimer, was obtained in a 73% yield (two steps). To our delight, a coupling of 22 with highly racemizable D -Dpg 7 (refs 30 , 31 ) afforded the desired pure tetrapeptide 23 , with no epimer, in a 79% yield (two steps) under condition A . The coupling of sterically hindered carboxylate 8 and tetrapeptide 24 afforded the desired pure pentapeptide 25 in a 51% yield (two steps). The removal of the Alloc group of protected pentapeptide 25 was performed using a solid-immobilized Pd catalyst in a batch reactor to facilitate the purification of polar pentapeptide. The subsequent coupling of highly racemizable D -Dpg 7 with pentapeptide 26 afforded the desired pure hexapeptide 2 with no epimer in a 70% yield (two steps). 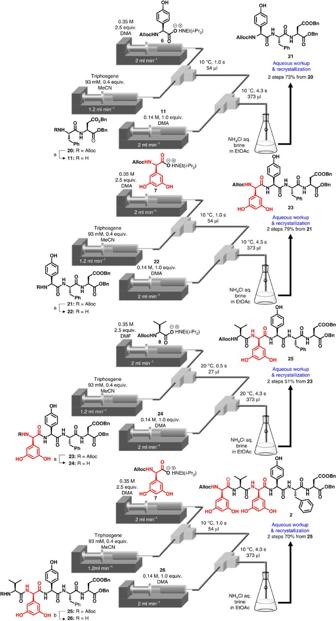Figure 3: Synthesis of C-terminal hexapeptide 2 using micro-flow amidation. Conditions: (a) Pd(PPh3)4, PhSiH3, CH2Cl2/MeOH, r.t., 1–1.5 h, batch. (b) PS-Ph3P-Pd, PhSiH3, CH2Cl2/MeOH/H2O, r.t., 1 h, batch. Figure 3: Synthesis of C-terminal hexapeptide 2 using micro-flow amidation. Conditions: ( a ) Pd(PPh 3 ) 4 , PhSiH 3 , CH 2 Cl 2 /MeOH, r.t., 1–1.5 h, batch. ( b ) PS-Ph 3 P-Pd, PhSiH 3 , CH 2 Cl 2 /MeOH/H 2 O, r.t., 1 h, batch. Full size image Synthesis of N-terminal heptapeptide 3 Synthesis of N-terminal heptapeptide 3 was performed based on the linear approach, as shown in Fig. 4 . The coupling of 9 with highly racemizable D -Dpg 7 under condition A caused a substantial generation of the undesired epimer (11%), whereas condition B afforded the desired peptide 27 in a 76% yield without severe racemization (1%). Dipeptide 14 was coupled with 6 under condition B to afford the desired tripeptide 28 in a 66% yield (two steps). The coupling of 29 with highly racemizable D -Dpg 7 was performed under condition B to afford tetrapeptide 30 in a 49% yield (two steps). The next coupling reaction of tetrapeptide 31 with 8 was performed to afford pentapeptide 32 in a 36% yield (two steps). In this reaction, 31% of the unreacted tetrapeptide 31 was recovered. The subsequent coupling of 33 with highly racemizable D -Dpg 7 under condition B using 5.0 equiv. of 7 , and 0.8 equiv. of triphosgene afforded the desired hexapeptide 34 in a 51% yield (two steps). The use of an excess amount of 7 and triphosgene was important for the return of a good yield. In this reaction, 34% of unreacted pentapeptide 33 was recovered. Hexapeptide 35 was coupled with 10b under condition B using 5.0 equiv. of 10b and 0.8 equiv. of triphosgene, and the subsequent preparative thin layer chromatography separation afforded the pure heptapeptide 3 with no epimer in a 25% yield (two steps). In this reaction, 24% of the unreacted 35 was recovered. In these reactions as well as in other amide bond formations, expensive Hpgs and Dpgs were recovered and reused. It should be noted that peptide chain elongation without severe racemization was achieved based on a linear approach that was considered impossible in feglymycin total synthesis. In addition, the coupling of racemizable amino acids usually requires low temperature and a long reaction time, whereas our developed process allowed rapid coupling (≤5.3 s). 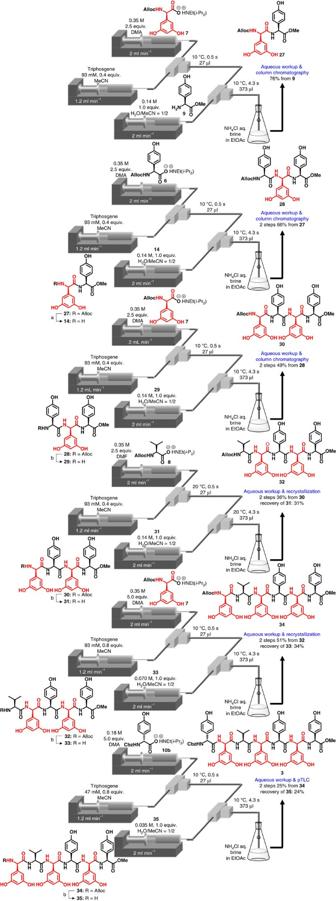Figure 4: Synthesis of N-terminal heptapeptide 3 using micro-flow amidation. Conditions: (a) Pd(PPh3)4, PhSiH3, CH2Cl2/MeOH/H2O, r.t., 40 min, batch. (b) PS-Ph3P-Pd, PhSiH3, CH2Cl2/MeOH/H2O, r.t., 1.5–2.5 h, batch. Figure 4: Synthesis of N-terminal heptapeptide 3 using micro-flow amidation. Conditions: ( a ) Pd(PPh 3 ) 4 , PhSiH 3 , CH 2 Cl 2 /MeOH/H 2 O, r.t., 40 min, batch. ( b ) PS-Ph 3 P-Pd, PhSiH 3 , CH 2 Cl 2 /MeOH/H 2 O, r.t., 1.5–2.5 h, batch. Full size image Total synthesis of feglymycin ( 1 ) Deprotection and coupling of hexapeptide 2 and heptapeptide 3 was performed in accordance with the Süssmuth group report ( Fig. 5 ). The structure of obtained feglymycin ( 1 ) was confirmed by 1 H and 13 C NMR, IR, and HRMS spectra, as well as by specific rotation. The observed spectra were consistent with the previously reported data [12] . 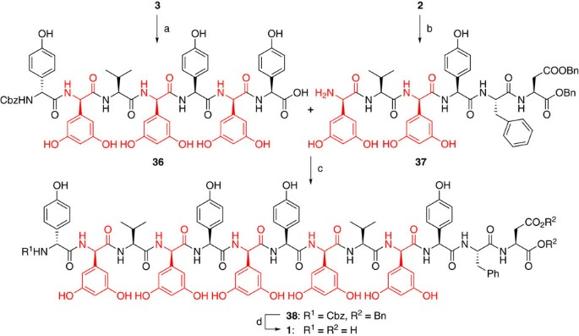Figure 5: Total synthesis of feglymycin (1). Conditions: (a) Me3SnOH, 1,2-dichloroethane; 85 °C, 3.5 h; (b) PS-Ph3P-Pd, PhSiH3, CH2Cl2/MeOH/H2O, r.t., 50 min; (c) DEPBT, NaHCO3, DMF, 0 °C, 24 h, then 25 °C, 11 h, 2 steps 44% from heptapeptide3. (d) H2, Pd/C, MeOH, r.t., 3 h, quant. Figure 5: Total synthesis of feglymycin (1). Conditions: ( a ) Me 3 SnOH, 1,2-dichloroethane; 85 °C, 3.5 h; ( b ) PS-Ph 3 P-Pd, PhSiH 3 , CH 2 Cl 2 /MeOH/H 2 O, r.t., 50 min; ( c ) DEPBT, NaHCO 3 , DMF, 0 °C, 24 h, then 25 °C, 11 h, 2 steps 44% from heptapeptide 3 . ( d ) H 2 , Pd/C, MeOH, r.t., 3 h, quant. Full size image In summary, we demonstrated a total synthesis of feglymycin based on a linear/convergent hybrid synthetic approach. Our originally developed micro-flow amide bond formation enabled the efficient preparation of hexapeptide 2 and heptapeptide 3 containing highly racemizable D -Dpgs based on a linear synthetic approach that was previously thought to be impossible. The developed synthetic approach will be useful for the rapid preparation of feglymycin analogues in the future. Our micro-flow amide bond formation uses triphosgene, and only emits CO 2 and HCl salt of DIEA. One of the advantages of using microreactors is the ease of scaling up. It should be possible to scale-up our developed process by either continuous operation or by a numbering-up of the microreactors. Our developed process will enable the practical preparation of biologically active oligopeptides containing highly racemizable amino acids. General NMR spectra were recorded on JEOL Model ECP-400 (400 MHz for 1 H, 100 MHz for 13 C) or Bruker Biospin AVANCE II 400 (400 MHz for 1 H, 100 MHz for 13 C), Bruker Biospin AVANCE III HD 500 (500 MHz for 1 H, 125 MHz for 13 C) instrument in the indicated solvent. Chemical shifts are reported in units of parts per million (p.p.m.) relative to the signal (0.00 p.p.m.) for internal tetramethylsilane for solutions in CDCl 3 (7.26 p.p.m. for 1 H, 77.0 p.p.m. for 13 C) or DMSO (2.50 p.p.m. for 1 H, 39.5 p.p.m. for 13 C). Multiplicities are reported by using the following abbreviations: s; singlet, d; doublet, t; triplet, q; quartet, m; multiplet, br; broad, J ; coupling constants in Hertz (Hz). IR spectra were recorded on Perkin-Elmer Spectrum One FT-IR spectrometer or JASCO FT/IR-4100. Only the strongest and/or structurally important peaks are reported as IR data given in cm −1 . Optical rotations were measured using a JASCO P-1020 or P-2200, Rudolph Research Analytical AUTOPOL IV. HRMS (ESI-TOF) were measured with a Bruker micrOTOF II. All reactions were monitored by thin-layer chromatography carried out on 0.25 mm E. Merck silica gel plates (60F-254) with ultraviolet light, visualized by 10% ethanolic phosphomolybdic acid or 0.5% ninhydrin n -butanol solution. Flash column chromatography was performed on Silica Gel 60 N purchased from Kanto Chemical Co or Silica Gel PSQ 60B purchased from Fuji Silysia Chemical LTD. Analytical HPLC was carried out on Shimadzu LC-10AT VP Liquid Chromatograph with a Shimadzu RID-10A Refractive Index Detector and a Shimadzu SPD-10A VP UV–vis Detector, Shimadzu SCL-10A VP System Controller. MeCN was dried using a Glass Contour. DIEA was distilled from ninhydrin and KOH. For HPLC analysis of 18a–c and 19a–c , see Supplementary Figs 2–7 , and for NMR spectra of synthesized compounds and analysis of 18a–c and 19a–c , see Supplementary Figs 8–45 . Data availability The authors declare that the data supporting the findings of this study are available within the article (and its Supplementary Information files). The data supporting the findings of this study are available from the authors upon reasonable request. How to cite this article: Fuse, S. et al . Total synthesis of feglymycin based on a linear/convergent hybrid approach using micro-flow amide bond formation. Nat. Commun. 7, 13491 doi: 10.1038/ncomms13491 (2016). Publisher’s note : Springer Nature remains neutral with regard to jurisdictional claims in published maps and institutional affiliations.